Low-grade chromosomal mosaicism in human somatic and embryonic stem cell populations Current knowledge on chromosomal mosaicism in human cell cultures is mostly based on cytogenetic banding methods. The recent development of high-resolution full-genome analysis methods applicable to single cells is providing new insights into genetic and cellular diversity. Here we study the genetic content of 92 individual human cells, including fibroblasts, amniocytes and embryonic stem cells (hESCs), using single-cell array-based comparative genomic hybridization (aCGH). We find that human somatic and embryonic stem cell cultures show significant fractions of cells carrying unique megabase-scale chromosomal abnormalities, forming genetic mosaics that could not have been detected by conventional cytogenetic methods. These findings are confirmed by studying seven clonal hESC sub-lines by aCGH. Furthermore, fluorescent in situ hybridisation reveals an increased instability of the subtelomeric regions in hESC as compared to somatic cells. This genetic heterogeneity may have an impact on experimental results and, in the case of hESC, on their potential clinical use. Human somatic tissues can contain a small fraction of aneuploid cells, forming a mosaic of euploid and aneuploid cells. In classic cytogenetics, clonal mosaicism refers to the situation in which a subpopulation of cells contains the same chromosomal aberration, as, for instance, in XX/XY mosaic individuals, while in non-clonal mosaicism the cells carry unique genomic abnormalities [1] , [2] . For somatic tissues, an important part of the knowledge on mosaicism has been obtained from studies using cytogenetic banding techniques, which provide information on whole chromosome copy number or large aberrations, and fluorescent in situ hybridization (FISH), studying a single locus. These studies have shown that the grade of mosaicism varies from tissue to tissue and the percentage of aneuploid cells increases with age, but provide limited insight on the occurrence of small genetic imbalances [2] , [3] , [4] , [5] . More recently, the group of Abyzov et al . [6] made use of the clonal nature of human-induced pluripotent stem cells (hiPSCs) to show that human skin fibroblasts are highly mosaic, with up to 30% of cells carrying copy number variants (CNVs). In the field of human pluripotent stem cell research, a large number of studies have shown that human embryonic stem cell (hESC) cultures are frequently taken over by chromosomally abnormal cells [7] , [8] , most probably because of a selective advantage caused by the chromosomal aberration [9] , [10] . Conversely, not much is known on how frequently hESC spontaneously mutate, either through abnormal chromosome segregation or by acquiring small amplifications or deletions, nor on the nature of these changes. In recent years, many groups have performed high-resolution screening of somatic cell populations [1] , [6] , [11] , [12] as well as hiPSC and hESC [7] , [8] and have reported de novo CNVs ranging from 10 kb to several Mb. It is important to bear in mind that these studies are based on the analysis of DNA from extractions from large numbers of cells, which only allows detection of CNVs if they are present in at least 5–10% of the cells [11] , [12] . In contrast, the recent development of new methods for the comprehensive study of the single cell genome [13] , [14] , [15] , [16] , epigenome [17] and transcriptome [18] is leading to a new understanding of cellular diversity. For instance, the study of single breast cancer cells revealed a significant number of de novo DNA copy number changes that appeared after only one cell cycle [15] and the analysis of large numbers of single cells has provided interesting insight in the evolution of genetically different cell populations within one tumour [14] , [15] , [16] . In the field of hiPSC, a recent study described low-grade mosaicism in neurons and differentiated hiPSCs at high resolution using array-based comparative genomic hybridization (aCGH) and single-cell sequencing [19] . In this study, we used single-cell aCGH, aCGH on clonal hESC lines and interphase FISH to investigate the occurrence of de novo CNVs in human somatic and embryonic stem cells. We find that both human somatic and embryonic stem cell cultures are genetically mosaic, with similar fractions of cells carrying unique gains and losses of chromosomal regions. On the other hand, FISH reveals that hESCs have a significantly increased instability of the subtelomeric regions as compared with somatic cells. These results show that both cell-type cultures show an important and differential genetic heterogeneity. Detection of genetic imbalances in single cells by aCGH To establish the sensitivity and resolution of our single-cell aCGH set-up, we used four cell lines carrying known chromosomal abnormalities. Amniocyte line A carried a derivative chromosome 5 (der(5)t(5;9)(p13.3;q33.3), amniocyte line B had a deletion of 5p15.33p15.1, amniocyte line C carried a trisomy 18, and hESC line VUB07 carried gains of 3q26.32q27.3 and of 20q11.21 (ref. 20 ). Details on the establishment of these lines and the identification and characterization of their genetic abnormalities can be found in the Methods section. First, we carried out aCGH on bulk DNA obtained from a large number of cells of the different lines, using the same platform as we used later for the single-cell analysis. This microarray has a lower probe density (hence resolution) than the oligonucleotide-based arrays used during the first characterization of the cell lines. In this setting, the imbalances found in amniocyte line A were covered by 32 probes on chromosome 5 and 17 on chromosome 9. For amniocyte line B, the loss of 5q15.33p15.1 was covered by 19 probes. The trisomy 18 in amniocyte line C represented 71 probes. For VUB07, while the gain in 3q26.32q27.3 represented seven probes, the gain of 20q11.21 was only covered by one probe, making the detection of this abnormality impossible using this specific platform, even on the DNA obtained from a large sample of cells. The results of these arrays are shown in Fig. 1 . 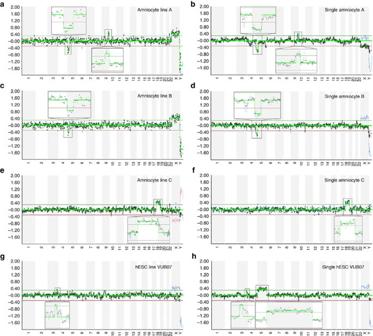Figure 1: Validation of single-cell aCGH platform. The aCGH plots in the left column present the results of bulk DNA analysis from whole-cell cultures. The right column contains examples of single-cell aCGH plots. (a,b) aCGH plots for amniocyte line A carrying a del(5)p13.3p15.33 and a dup(9)q33.3q34.3. (c,d) aCGH plots for amniocyte line B carrying a del(5)p15.33p15.1. (e,f) aCGH plots for amniocyte line C carrying a trisomy 18. (g,h) aCGH plots for hESC line VUB07 carrying a dup(3)q26.33q27.3. All samples are arrayed against female and male reference DNAs, and the aCGH plots displayed here show the combined results of the two tests, except fora,b,f, which were only arrayed against a male reference. Zoom-in boxes illustrate called CNVs compared with the reference DNA. The thick green line indicates significant deviations from the average log-2 ratio and is used for CNV calling. A green and a red horizontal guideline indicate a log-2 ratio of 0.3 and −0.3, respectively, although the log-2 ratio threshold for calling gains and losses of genetic material were 0.31 and −0.45, respectively. A blue and red line following the log-2 ratios of the different probes indicate relative log-2 ratios compared with the male (blue) and female (red) reference DNA. Figure 1: Validation of single-cell aCGH platform. The aCGH plots in the left column present the results of bulk DNA analysis from whole-cell cultures. The right column contains examples of single-cell aCGH plots. ( a , b ) aCGH plots for amniocyte line A carrying a del(5)p13.3p15.33 and a dup(9)q33.3q34.3. ( c , d ) aCGH plots for amniocyte line B carrying a del(5)p15.33p15.1. ( e , f ) aCGH plots for amniocyte line C carrying a trisomy 18. ( g , h ) aCGH plots for hESC line VUB07 carrying a dup(3)q26.33q27.3. All samples are arrayed against female and male reference DNAs, and the aCGH plots displayed here show the combined results of the two tests, except for a , b , f , which were only arrayed against a male reference. Zoom-in boxes illustrate called CNVs compared with the reference DNA. The thick green line indicates significant deviations from the average log-2 ratio and is used for CNV calling. A green and a red horizontal guideline indicate a log-2 ratio of 0.3 and −0.3, respectively, although the log-2 ratio threshold for calling gains and losses of genetic material were 0.31 and −0.45, respectively. A blue and red line following the log-2 ratios of the different probes indicate relative log-2 ratios compared with the male (blue) and female (red) reference DNA. Full size image Next, we carried out single-cell aCGH for eight amniocytes of line A, two amniocytes of line B, two amniocytes of line C and three single hESCs of VUB07. Examples of the aCGH plots are shown in Fig. 1 . After data processing, only arrays with s.d. ≤0.15, >80% included clones, signal-to-background ratio >3 and derivative log-ratio <0.2 were considered for further analysis. For the single-cell aCGH set-up using the 24sure v3.0 platform, samples were in silico compared with two reference DNA sets (male and female, respectively), and aberrant calls were only considered if present when compared with both references. We found that a threshold of 0.31 for the log2 ratio of gains of chromosomal content, and −0.45 for loss of chromosomal content, resulted in the consistent call of the sex mismatches and allowed us to detect 18 out of 23 expected abnormalities in the control single cells, with only one extra positive call. These thresholds were also in line with the manufacturer’s guidelines and the theoretical log2 thresholds (0.3 for gain, −0.45 for loss). In addition, since only arrays with a s.d. ≤0.15 were considered for further analysis, every called abnormality had a mean log2 ratio of more than twofold the s.d. of the array itself. While the expected chromosome losses were all reliably detected, the duplication of 9q33.3q34.3 in amniocyte line A was only called in three out of eight single cells. This under-calling of small chromosome gains is due to the conservative calling approach. For example, in amniocyte A07 the 9q33.3q34.3 amplification is visible when analysing the raw data (see Supplementary Fig. 1i ); however, the log2 ratio of the abnormal region remains below the cutoff value of 0.31. We deemed preferable to have an increased false-negative rate to a false-positive rate, which would have been the consequence of lowering the threshold for the calling of gains. To define the resolution of our single-cell aCGH set-up, we used the smallest abnormality that we were able to consistently call in our control cells: the gain in 3q26.32q27.3 in VUB07. This abnormality spanned seven consecutive clones, which we set as the minimum number of clones for an abnormality to be called aberrant in this specific aCGH setting. Here again, it is possible that this approach resulted in an under-calling of abnormalities. We found several segments of less than seven consecutive clones that reached the cutoff log2 ratios but were not called for the sake of consistency (for example, VUB02 P59 03, where five clones on 19p12p13.11 reach a log2 ratio of 0.332, see Supplementary Fig. 2e ). The average spacing of the microarray probes over the chromosomes was ~1 Mb, but given that the probe density varied depending on the chromosomal region, we are unable to define a resolution of our setup in Mb. Next, we carried out single-cell aCGH for 17 single human fibroblasts and 60 single cells of two different passages of the hESC line VUB02 (passages 59 and 351), along with DNA samples extracted from whole cultures of the same cell lines. Again, only arrays with s.d. ≤0.15, >80% included clones, signal-to-background ratio >3 and derivative log-ratio <0.2 were considered for further analysis. Abnormalities were called based on the thresholds previously set and were cross-checked for their presence when comparing with both male and female reference DNAs, leading to the exclusion of one call in cell 14 of VUB02 P59 showing an abnormality for chromosome 1 that was only present compared with the female reference DNA ( Supplementary Fig. 2o , red square). The sample was tested again with a different batch of reference DNA, and the false-positive aberration dropped below threshold, confirming the correctness of the negative call ( Supplementary Fig. 2p , red square). We also found a recurrent segmental amplification Xq13.2q22.1, which proved to be inconsistent after repeated arraying of the same sample (for example, Supplementary Fig. 2o and 2p, purple squares). We deduced that this was because of inconsistencies in the reference DNA, and we excluded the sex chromosomes from further analysis for segmental abnormalities. Finally, seven of the samples that showed an aberrant genomic content were re-arrayed, four of which with a dye-swop (Cy3-labelled in the second array if in the first test they were Cy5-labelled, and vice versa ). Reassuringly, only those abnormalities that matched the cutoff values we initially set were detected in both experiments, and no new abnormalities appeared. The only exception was the duplication of 19p13.3q13.11 in cell 05 of VUB02 passage 351, which remained undetectable after re-arraying. This may be explained by the fact that this abnormality involves chromosome 19, which is known to be a problematic region for CGH, probably because of its high GC content [21] . Four aberrations were called with slightly different breakpoints (an example is the deletion on chromosome 3q in VUB02 passage 59 cell 15). It is clear that one of the main bottlenecks in single-cell genomics is the inability to validate the results of the analysis of one specific cell by a second method. This makes it necessary to rely on the validation of the methodology using a control cell population with known genetic abnormalities. From our results, and that of other researchers, it is obvious that there are no such uniform cell lines, making the establishment of false-positive rates impossible. In our study, we chose to use a conservative calling approach, to minimize the false-positive rates but likely leading to an underestimation of the frequency of small CNVs. A second difficulty is that single-cell aCGH requires a step of whole-genome amplification (WGA). Over the years, many methods for WGA have been developed, each of them with their strengths and weaknesses [22] , [23] . Mainly, WGA methods differ in their yields and, more importantly, in their amplification bias. Nonlinear amplification of regions of the DNA can lead to the detection of false CNVs. For this study, we used a linker-adapter-mediated PCR-based system for the WGA: the Sureplex Amplification System. This method is known to perform well for the linear amplification of single cells. It generates fragments from 100 to 1,000 base pairs, with an average of 400 basepairs [22] , although it only amplifies a representation of the genome [23] . Since the abnormalities we are calling are in the Mb range, this minimizes the chance for a preferential over- or under-amplified fragment to be misinterpreted as a CNV. Furthermore, we used an aCGH platform and a raw data normalization pipeline that have been specifically tailored to this WGA method by the manufacturer. Nonetheless, it is clear that there are some technical variabilities between experiments, as reflected by the (small) differences in breakpoints of CNVs after analysing twice the same WGA product, or the inability of detecting 100% of the expected segmental abnormalities in the control cells when using a fixed log2 threshold. De novo CNVs in individual somatic and embryonic stem cells While the analysis of the bulk DNA samples only showed the previously known chromosomal abnormalities in the amniocytes, and a normal genetic content for the fibroblast samples and both passages of the hESC, the single-cell aCGH results revealed de novo CNVs in all cell types. Examples of single cells carrying de novo CNVs can be found in Fig. 2 , a complete overview of the genetic content of all samples can be found in Supplementary Table 1 and all aCGH plots are shown in Supplementary Figs 1–3 . 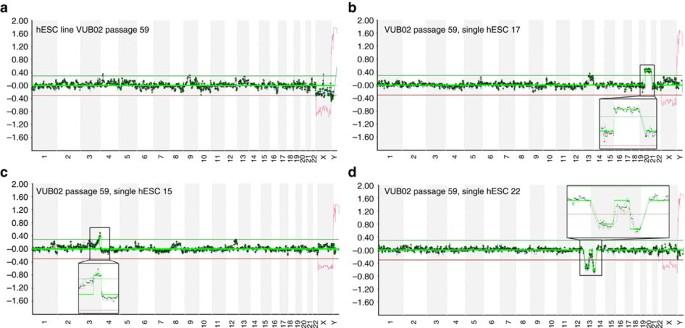Figure 2: aCGH plots of single cells showing unique CNVs. (a) Bulk DNA sample of VUB02 passage 59, showing no genomic aberrations. (b) VUB02 passage 59 single cell 17 carrying a trisomy 20. (c) VUB02 P59 single cell 15 carrying a duplication of chromosome 3q26.33q29. (d) VUB02 passage 59 single cell 22 carrying a deletion of chromosomes 13p12.11q14.3 and 13q32.1q34. All samples are arrayed against female and male reference DNA, and the aCGH plots displayed here show the combined results of the two tests. Zoom-in boxes illustrate called CNVs compared with the reference DNA. The thick green line indicates significant deviations from the average log2 ratio and is used for CNV calling. A green and a red horizontal guideline indicate a log2 ratio of 0.3 and −0.3, respectively, although the log2 ratio threshold for calling gains and losses of genetic material were 0.31 and −0.45, respectively. A blue and red line following the log2 ratios of the different probes indicate relative log2 ratios compared with the male (blue) and female (red) reference DNA. Figure 2: aCGH plots of single cells showing unique CNVs. ( a ) Bulk DNA sample of VUB02 passage 59, showing no genomic aberrations. ( b ) VUB02 passage 59 single cell 17 carrying a trisomy 20. ( c ) VUB02 P59 single cell 15 carrying a duplication of chromosome 3q26.33q29. ( d ) VUB02 passage 59 single cell 22 carrying a deletion of chromosomes 13p12.11q14.3 and 13q32.1q34. All samples are arrayed against female and male reference DNA, and the aCGH plots displayed here show the combined results of the two tests. Zoom-in boxes illustrate called CNVs compared with the reference DNA. The thick green line indicates significant deviations from the average log2 ratio and is used for CNV calling. A green and a red horizontal guideline indicate a log2 ratio of 0.3 and −0.3, respectively, although the log2 ratio threshold for calling gains and losses of genetic material were 0.31 and −0.45, respectively. A blue and red line following the log2 ratios of the different probes indicate relative log2 ratios compared with the male (blue) and female (red) reference DNA. Full size image The ideograms in Fig. 3a,b show the de novo CNVs found in hESC (both passages of VUB02) and somatic cells (amniocytes and fibroblasts), respectively. Table 1 summarizes the different types of chromosomal aberrations per cell type. In passages 59 and 351 of hESC line VUB02, five (17.2%) and one (3.2%) of the cells, respectively, carried at least one genetic imbalance. For human somatic cells, three fibroblasts (17.6%) and one amniocyte (8.3%) showed CNVs that were not detected at the level of the whole culture. None of the frequencies of de novo CNVs was found to be statistically different between cell types (Fisher’s exact test). In total, we detected 14 segmental genetic imbalances between 4.36 and 44 Mb in size, with an average of 21.1 and 21.0 Mb for the hESC and somatic cell types, respectively. Eleven (78.6%) of those CNVs spanned up to the telomeric region. 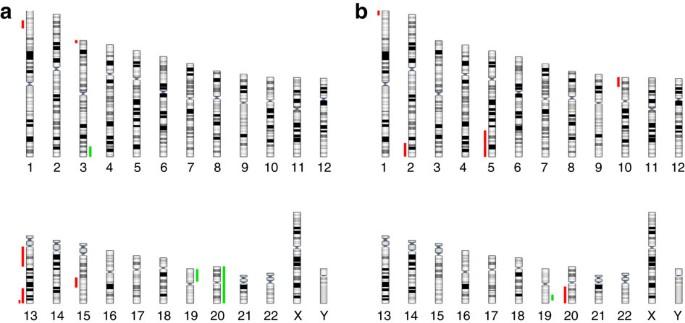Figure 3: aCGH analysis of hESC, amniocytes and fibroblasts. (a,b) Ideogram showing allde novocopy number changes found in 60 hESCs of two different passages of VUB02 (a) and in 17 cultured human fibroblasts and 12 amniocytes (b). Gains are marked in green, losses in red. The triploid VUB02 passage 59, single cell 10 is not included in the ideogram. Figure 3: aCGH analysis of hESC, amniocytes and fibroblasts. ( a , b ) Ideogram showing all de novo copy number changes found in 60 hESCs of two different passages of VUB02 ( a ) and in 17 cultured human fibroblasts and 12 amniocytes ( b ). Gains are marked in green, losses in red. The triploid VUB02 passage 59, single cell 10 is not included in the ideogram. Full size image Table 1 aCGH analysis of hESC, amniocytes and fibroblasts. Full size table The fact that we did not detect any of the abnormalities found at the single-cell level in the DNA extracted from the whole-culture dish, and that none of the cells of a same population showed the same abnormality, suggests that they are either unique to each cell or belong to clones with very low frequencies in the culture. The size, nature and frequencies of these segmental CNVs are comparable to the abnormalities recently reported in fibroblasts [6] , differentiated hiPSC and neurons studied using aCGH and single-cell sequencing [19] . Remarkably, we only found full chromosome aneuploidy in two hESCs and none in the somatic cells: one hESC contained a trisomy 20 and one was triploid. This is in line with previously reported aneuploidy rates in amniocytes studied by banding methods [2] and hESC studied by metaphase CGH [24] . On the other hand, they are in contrast with the high percentages of non-clonal aneuploidy reported by studies using FISH on cultured somatic cells [3] , [4] and hESC [25] , [26] . It is likely that the use of different techniques is the cause of these discrepancies. Interphase FISH reveals subtelomeric instability in hESC To address the differences in nature and frequency of the CNVs between our data and the high frequencies of whole-chromosome aneuploidies found by studies using FISH [3] , [4] , [25] , [26] , we analysed the amniocyte, fibroblast and hESC lines by FISH on interphase nuclei for two randomly selected chromosomes. We used probes for the centromere and both subtelomeric regions of chromosomes 1 and 18, allowing us to distinguish between full chromosome aneuploidy and segmental gains or losses of chromosome arms or subtelomeric regions. From the results summarized in Table 2 it can be appreciated that, in line with the aCGH data, we find few to no aneuploidies for the hESC and the somatic cells, while gain and loss of a subtelomeric region occurred repeatedly, with a significant higher abnormal fraction in hESC compared with the somatic cells (Fisher’s exact test, P ≤0.05 for both chromosomes). Table 2 FISH analysis of hESC, amniocytes and fibroblasts. Full size table Next, we evaluated the FISH on hESC by looking only at the centromeric probe of chromosome 18, to call for euploidy or aneuploidy. In this case, we found that out of 931 interphases, 22 seemed to carry a monosomy (2.3%) and one a trisomy 18 (0.1%). Extrapolated to the 23 chromosome pairs, this would amount to about 55% aneuploidy, which is comparable to the data previously reported [25] , [26] . However, a cross-check of the same spreads by taking the telomeric probes into account, and thus using three probes per chromosome, showed that only three of these whole-chromosome aneuploidy calls were correct. Unlike in somatic cells, we found that in hESC the centromeric probes frequently showed overlapping signals, resulting in a false-positive monosomy call if only this probe was considered (an example can be found in Fig. 4 ). Hence, the use of different FISH probes in the different studies, the extrapolation of the information of a single locus to whole-chromosome abnormality and to 23 pairs and the fact that probably some cells carry more than one abnormalities rather than each cell one, may be the reason for at least part of the differences between studies. 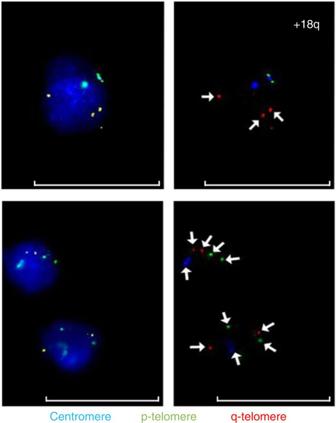Figure 4: FISH analysis of hESC, amniocytes and fibroblasts. Example images for FISH analysis of VUB02 passage 351 with 4',6-diamidino-2-phenylindole (DAPI; left images) and without DAPI (right images). Centromeres are labelled in aqua, p-telomeres in green and q-telomeres in orange. The top two frames show a hESC with an 18q amplification. The lower frames show two examples of cells that could be scored as monosomic if only the centromeric probe would be taken into account. The presence of all four telomeres suggests that the centromeric probes are overlapping. White scale bars represent 25 μm. Figure 4: FISH analysis of hESC, amniocytes and fibroblasts. Example images for FISH analysis of VUB02 passage 351 with 4',6-diamidino-2-phenylindole (DAPI; left images) and without DAPI (right images). Centromeres are labelled in aqua, p-telomeres in green and q-telomeres in orange. The top two frames show a hESC with an 18q amplification. The lower frames show two examples of cells that could be scored as monosomic if only the centromeric probe would be taken into account. The presence of all four telomeres suggests that the centromeric probes are overlapping. White scale bars represent 25 μm. Full size image On the other hand, in hESC, the frequencies of segmental gains or losses revealed using FISH (39.1–46% when extrapolated to 23 chromosome pairs) do not correlate with the frequencies of segmental abnormalities spanning the telomeric regions seen by single-cell aCGH (10.0%). An important point to bear in mind is that the FISH probes for the telomeres target a region outside of the coverage of the microarray platform used in this study. Therefore, the FISH is able to reveal abnormalities of the subtelomeres that the microarrays are not. It is possible that the excess of abnormalities measured using FISH reflects an increased instability of the subtelomeric regions, as seen in human tumour cells and mouse ESC. These cells appear to be very prone to misrepair of double-stranded breaks occurring close to the telomeres, leading to copy number changes and chromosomal rearrangements [27] , [28] . Subcloning of hESC line VUB02 reveals unique CNVs Finally, we aimed at investigating whether the abnormalities we found in the individual cells could be stably transmitted to a clonal population. For this, we created clonal hESC lines, originating from single hESC. We dissociated a few colonies of VUB02 passage 351 to single cells and plated them on mouse feeder layers (see Methods). We individually expanded seven of the new colonies for three passages, and extracted DNA from each culture. Using the 4 × 44 k Oligo-based aCGH platform from Agilent, providing a higher resolution than the arrays used for the single-cell aCGH, we screened the sublines for unique CNVs. In all sublines we found the gain of 20q11.21, known to be present at this passage of VUB02, and the losses of the polymorphic CNVs at 3p25.2p25.2 and 22q13.31q13.31, forming a fingerprint of the original cell line (see Table 3 ). Table 3 aCGH analysis of clonal hESC sublines. Full size table In five sublines, we found unique CNVs, and in clonal subline 1 we found a 9.7 Mb amplification of chromosome 12p13.31p13.33 and a deletion of 2.4 Mb in chromosome 13q34 ( Fig. 5a,b ). These segmental aberrations both span the telomere, similar to 78.6% of the segmental aberrations detected with the single-cell aCGH. Remarkably, the amplification of 12p13.31p13.33 includes the gene NANOG , which plays a key role in the control of pluripotency. 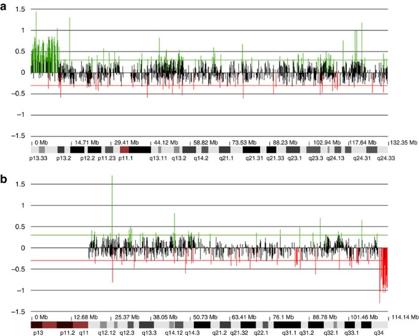Figure 5: aCGH analysis of clonal hESC sublines. Array-based CGH plots of chromosome 12 (a) and 13 (b) of clonal subline 1, showing a 12p13.31p13.33 amplification and a 3q34 deletion. The green bars indicate amplifications compared with the reference set, red bars indicate deletions compared with the reference set. Figure 5: aCGH analysis of clonal hESC sublines. Array-based CGH plots of chromosome 12 ( a ) and 13 ( b ) of clonal subline 1, showing a 12p13.31p13.33 amplification and a 3q34 deletion. The green bars indicate amplifications compared with the reference set, red bars indicate deletions compared with the reference set. Full size image The smallest CNVs detected in this part of the study were below the resolution of the single-cell aCGH platform. Of the two largest CNVs, the deletion in chromosome 13q34 would be covered by five probes of the single-cell aCGH platform and the 12p13.31p13.33 amplification would span 11 probes, making only the latter falling within the resolution of this set-up. Since each clonal subline represents the genetic content of one single hESC of the original culture, this result can be seen as a confirmation of the low-grade mosaicism detected with the single-cell aCGH above. By combining three independent approaches we detected low-grade de novo CNVs in hESC, fibroblasts and amniocytes. Interestingly, the nature of those abnormalities is different than previously thought. Here we describe mainly segmental chromosomal abnormalities, of which most spanned the telomeres, while whole-chromosome aneuploidies were detected only sporadically. Furthermore, hESC seem to undergo subtelomeric instability at a higher frequency than somatic cells. This is distinctive from the majority of previous studies that focused on analysing single cells, which lacked the resolution to detect the majority of the CNVs described here [3] , [4] , [25] , [26] . As these CNVs are present at very low frequencies in the culture, they also could not be detected using the straight-forward analysis of pooled DNA, as used by most studies for high-resolution screening of cell lines. To get around this, Abyzov et al . [6] derived hiPSC lines from skin biopsies to clonally amplify the genetic content of single fibroblasts and described low-frequency kilo-base scale CNVs unique to each subclone. This is indicative for low-grade mosaicism in the original fibroblasts; however, the CNVs described by Abyzov et al . [6] are considerably smaller than the CNVs described in this study. A very recent publication reports genetic mosaicism of megabase-scale CNVs in differentiated hiPSC, cultured fibroblasts and neurons using various high-resolution single-cell genomics [19] . The reported CNVs are very similar to our data, with predominantly segmental CNVs of a comparable size range, and low frequencies of aneuploidies. The combination of both studies provides solid proof that cultured cells exhibit high frequencies of genetic aberrations. Even so, this is, to our knowledge, the first study to describe this kind of genetic mosaicism in hESC cultures. Because of the lack of a genetically uniform cell line to be used as a negative control, we are unable to define the false-positive rate caused by technical noise. This makes it challenging to compare the frequencies of CNVs in different populations; however, with our conservative calling approach we limit the risk for over-calling to a minimum. Comparing the abnormal fractions in both passages of VUB02 using aCGH, we could not find a statistically significant difference, which was in line with the FISH results. Nevertheless, it would not be unrealistic to suggest that the degree of low-grade mosaicism can differ between cell cultures, given their differences in metabolism, culture conditions, proneness to DNA damage, and so on. In addition, for the different passages of hESC, culture adaptation could increase the cell’s capacity to cope with replication stress induced by suboptimal culture conditions, lowering the DNA damage and the need for DNA (mis-) repair. Further study, including larger numbers of single cells, could clarify this further. Remarkably, despite having almost 300 passages of difference, we could not detect the clonal amplification of any CNV in the pooled DNA samples of VUB02 within the size range of the CNVs detected with the single-cell aCGH. Most of the de novo CVNs detected with the single-cell aCGH or the FISH are deletions; however, the majority of clonally amplified genomic aberrations previously described in hECS are amplifications [29] . This might indicate that most of the CNVs are selected against due to deleterious effects for the cells. However, VUB02 passage 351 does contain the 20q11.21 amplification, which is known to provide a survival advantage [9] , [10] . This indicates that CNVs that start as a single-cell event can clonally take over the culture. In addition it is likely that the higher the frequency of those de novo CNVs the higher the chance for a CNV to occur that will clonally expand. The cause of these large CNVs remains unclear. The high frequency of segmental aberrations found in this study implies that both cultured somatic cells and hESCs frequently undergo DNA breaks, which are incorrectly or not repaired in a significant number of cases. Three quarters of the abnormalities spanned the telomeric regions, as previously found in cells undergoing replication stress [30] . Taken together, this suggests that the majority of the detected CNVs may have originated by replication fork collapse, eventually followed by breakage-induced replication. This could be explained by suboptimal culture conditions as the driving mechanism behind the non-clonal or low-grade mosaicism, although this should be subject to further research. In conclusion, both hESC and somatic cells frequently carry an imbalanced chromosomal content, leading to highly mosaic cultures. While the frequency of these abnormalities appears to be similar in both cell types, hESC shows a remarkably higher frequency of subtelomeric aberrations. The impact of the genetic heterogeneity on experimental results or, in the case of hESC, their potential clinical use, remains to be elucidated. Unravelling the driving mechanism behind these genetic mosaics would substantially contribute to all research based on in vitro cell culture. Cell lines and culture Normal dermal human fibroblasts (ATCC, Molsheim, France), hereafter called fibroblasts, were cultured in mouse embryonic fibroblast (MEF) medium (88% Dulbecco’s Modified Eagle Medium (DMEM), 10% fetal calf serum, 1% Glutamax and 1% nonessential amino acids) and harvested with 0.05% Trypsin/EDTA (all products provided by Life Technologies, Gent, Belgium). Amniocyte cultures were established and characterized by the ISO 15189 Laboratory of the Centre for Medical Genetics, Universitair Ziekenhuis Brussel (University Hospital Brussels, Belgium). They were kept in CHANG Medium C (Irvine Scientific, Newtownmountkennedy, Ireland) and harvested with 0.05% Trypsin/EDTA (all products provided by Life Technologies). G-banding of 20 metaphase spreads showed that amniocyte line A carried a derivative chromosome 5 (46,XX,der(5)t(5;9)(p13.3;q33.3)). Oligonucleotide-based comparative genomic hybridization (aCGH) showed a loss of 5p13.3p15.33 and a gain of 9q33.3q34.3. This was confirmed with FISH using subtelomeric probes for 5p and 9q. G-banding of 17 metaphase spreads of amniocyte line B showed that the line carried a deletion of 5p15 (46,XX,del(5)p15). This was confirmed using FISH with a subtelomeric probe for 5p. G-banding on 20 metaphase spreads showed that the karyotype of amniocyte line C was 47,XY,+18. VUB02 and VUB07 were derived and cultured as previously described [31] and are available upon request. Briefly, hESC colonies were grown on inactivated MEF feeder layers at 37 °C in 5% CO 2 , using a standard hESC medium: KnockOutTM-DMEM containing 20% KnockOutTM serum replacement (SR, Invitrogen, Carlsbad, USA), 2 mM-glutamine (Invitrogen), 1% non-essential amino acids (Invitrogen), 0.1 mM β-mercapto-ethanol (Sigma-Aldrich, Schnelldorf, Germany), penicillin/streptomycin 100 U ml −l (Invitrogen) and 4 ng ml −1 human recombinant basic fibroblast growth factor (Invitrogen). hESC colonies were passaged in clumps by mechanical slicing every 5–6 days. All hESC lines were characterized using aCGH, initially using in-house arrays from the Nucleomics Core (VIB, K.U. Leuven) [20] and later using the 4 × 44 K Human Genome array as described in the section below. For the aCGH using the in-house arrays 300 ng of test and reference DNA samples were labelled by random primer labelling (BioPrime Array CGH Genomic Labelling System, Invitrogen) using Cy5- and Cy3-labelled dCTPs (GE Healthcare, Buckinghamshire, UK), respectively. The labelled DNA was combined with 150 μg of Cot-1 DNA (human Cot-1 DNA; Invitrogen), followed by ethanol precipitation and resuspension in 20 μl hybridization buffer (50% formamide, 10% dextran sulfate, 0.1% Tween-20, 2 × SSC and 10 mM Tris-HCl, pH 7.5). The slide was blocked for an hour with 16.6 μg Cot-1 DNA and 100 μg salmon testis DNA (Sigma Aldrich) dissolved in 15 μl hybridization buffer containing 200 μg yeast tRNA (Invitrogen). Slides were hybridized in a humid chamber at 37 °C for 24–72 h. Following hybridization and washing of the slides, the arrays were scanned using an Agilent dual laser DNA microarray scanner G2566AA (Agilent Technologies, Palo Alto, CA, USA). The scan images were processed with the Agilent Feature Extraction Software v9.5 and the final steps of data analysis were performed using Excel (Microsoft Corporation, Redmond, WA, USA). Subline A of VUB02 had a normal genetic content (in this work, passage 59), while subline B (here at passage 351) carried a gain of 20q11.21. The subline of VUB07 used in this study was known to carry a gain of 3q26.32q27.3 and of 20q11.21. For the creation of the clonal sublines, hESCs were pre-incubated with 10 μM of ROCK inhibitor, Y-27632 (Y05031MG, Sigma-Aldrich, water soluble) for 1 h before detaching from the feeder layer. Single hESC was then collected using non-enzymatic cell dissociation solution (C5914, Sigma-Aldrich). The cell suspension was passed through a 40-μm cell strainer (BD Falcon, BD Biosciences, 9320 Erembodegem, Belgium) to remove remaining clumps and was pelleted using centrifugation at 115 × g for 5 min. The cell pellet was resuspended in standard hESC medium. Approximately 100 single cells were plated on inactivated MEF feeder layers and cultured under standard conditions for 10–12 days. Ten clones (single hESC colonies) were selected and further cultured separately for three passages before DNA extraction. Single-cell aCGH hESC colonies were dissociated into single cells using non-enzymatic cell dissociation solution (Sigma-Aldrich). Individual hESCs were manually washed by serial transfer in drops of phosphate-buffered saline (Cell Signaling Technologies) with 0.1% polyvinylpyrrollidone and collected into sterile PCR tubes as previously described [32] , [33] . The cell’s DNA was amplified using the SurePlex DNA Amplification System (BlueGnome, Cambridge, UK), a ligation-mediated PCR-based technique, according to the manufacturer’s instructions. The Sureplex WGA procedure consists of three steps: extraction and fragmentation of the genomic DNA of the isolated cells to fragments in the range of a few hundred basepairs, ligation of specific adaptor sequences to both ends of the fragments and a subsequent amplification reaction by PCR using the flanking universal priming sites contained in the adaptors. This system is widely used in the clinical setting for pre-implantation genetic diagnosis starting from single-cell material [34] and, although it only amplifies a representation of the genome, has a relatively low allele-dropout rate and amplification bias [22] , [23] . In this study, we used the 24sure array platform (BlueGnome). It consists of DNA probes derived from bacterial artificial chromosomes (BAC) clones from the Roswell Park (RP-nomenclature) human genome collection. The BAC clones are PCR-amplified and immobilized on microarray slides; 2,909 unique probes are spotted and each clone is spotted in duplicate. The array has an average but variable coverage spacing of 1 Mb on the human genome. aCGH was carried out according to the BlueGnome 24sure protocol, without modifications ( http://www.cambridgebluegnome.com ). Briefly, DNA samples (both genomic DNA as Sureplex amplified single cells) were labelled with Cy3 or Cy5 at 37 °C for 4 h using the labelling kit provided by the manufacturer. We used a dual-channel set-up, with male and female reference DNA labelled once with each label for each run; the samples were compared in silico with the male and female reference DNAs. The reference DNA used in these experiments is the SureRef reference DNA (male and female), which is an amplified genomic DNA, and is provided by the same manufacturer. After combination with Cot-1 DNA and ethanol precipitation at −80 °C for 20 min, DNA was resuspended in hybridization buffer for 10 min at 75 °C. Overnight hybridization at 47 °C in 50% formamide/2% saline-sodium citrate-humidified chambers was followed by the standard 24sure washing protocol (buffers and protocol provided by BlueGnome). An Agilent dual laser DNA microarray scanner G2566AA was used for scanning the slides. aCGH data analysis TIFF files were imported and processed using BlueFuse Multi 3.1 (BlueGnome). Only arrays with s.d. ≤0.15, >80% included clones, signal-to-background ratio >3 and derivative log-ratio <0.2 were considered for further analysis. The log2 ratios are normalized with BlueFuse Multi 3.1 for systematic noise by taking into account variations from the zero-line when reference DNA was hybridized to itself. In addition, an intensity bias correction was performed to correct for differences in laser power and sensitivity for the different labels, and GC base content bias correction for differences in hybridization efficiency. Each BAC probe was spotted twice per sample and was only included if the log2 ratio difference between them was <0.1 s.d. of the array. The average over the replicates was chosen as value for that locus if included. Finally, the BlueFuse Multi 3.1 programme reduced the background noise by smoothing the log2 ratios with a window size of three consecutive clones. The software provides scatterplots of both the raw and normalized data, which were used for visual inspection of the results. Examples of scatterplots of the normalized data can be found in Supplementary Figs 1–3 . Next, the normalized log2 ratios were exported from the BlueFuse Multi 3.1 software and analysed using a web-based implementation of the Circular Binary Segmentation (CBS) algorithm ( http://compbio.med.harvard.edu/CGHweb ). This algorithm identified chromosome regions of similar log2 ratio, with a probability of 95% ( α =0.05) and a threshold log2 ratio of 0.3. For more details on the CBS algorithm see Olshen et al . [35] The average log2 ratios provided using the CBS were used to call the chromosomal abnormalities, using the thresholds established during the validation of the platform. 4 × 44 K human genome aCGH We used the protocol for oligo arrays as implemented in the ISO 15189 Laboratorium of the Centre for Medical Genetics, Universitair Ziekenhuis Brussel (University Hospital Brussels), based on the protocol provided by Agilent Technologies. In brief, the DNA was purified using Amicon Ultra 30 K centrifugal filter tubes (Merck Chemicals, Overijse, Belgium). A total of 400 ng of DNA was combined with 26.7 μl random primers (BioPrime aCGH Labeling module, Life Technologies), 1.3 μl NaCl and diluted to a volume of 57.7 μl, followed by 15-min denaturation at 98 °C. The samples were labelled with Cy3 while the reference DNA (Promega, Leiden, Netherlands) was labelled with Cy5, with an overnight incubation at 37 °C. Ethanol-precipitated samples were then dissolved in 42 μl TE-buffer (Promega) and mixed at 900 r.p.m. for 3 h at 42 °C. After the addition of Cot-1 DNA (Life Technologies), Blocking Agent and hybridization buffer (Agilent Technologies), samples were denaturated at 95 °C for 3 min and incubated at 37 °C for 30 min. Afterwards, the samples are hybridized on the microarray slide (4 × 44 K Human Genome CGH Microarray, Agilent Technologies) for 24-h incubation at 65 °C. This array contains 42,494 probes per samples, with an overall spacing of 43 and 24 kB in Refseq genes. Slides were washed with Oligo Wash Buffer 1 for 5 min at room temperature and in Oligo Wash buffer 2 at 37 °C for 1 min (Agilent Technologies), and afterwards with Stabilization and Drying solution for 1 min (Agilent Technologies) and for 30 s with acetonitrile (Sigma-Aldrich). Scanning of the slides was performed using an Agilent dual laser DNA microarray scanner G2566AA. After completion of the scan, the TIFF files were analysed using the workflow used for clinical analysis of the oligo-aCGH data, as implemented in the ISO 15189 Laboratory of the Centre for Medical Genetics, Universitair Ziekenhuis Brussel (University Hospital Brussels). Only arrays with a s.d. ≤0.20, signal intensity >50, background noise <5 and a derivative log-ratio <0.2 were considered for further analysis. The data were extracted using the Agilent Feature Extraction software and analysed with the ‘ArrayCGHbase’ analysis platform ( http://medgen.ugent.be/arrayCGHbasecmgg/ ) [36] . Cutoff values were set at three consecutive probes with an average log2 ratio over 0.3 for gains of genetic material and three consecutive clones with an average log2 ratio of −0.45 for loss of genetic material. FISH FISH was performed following the manufacturer’s instructions using Telvysion 1p, Telvysion 1q, Vysis CEP 18 probes, Telvysion 18p, Telvysion 18q (Abbott Molecular) for the telomeres of chromosome 1 and 18 and the centromere of chromosome 18. The probe for centromere 1 was not included because of the overlap in the labelling. Briefly, cells were fixed with carnoy’s fixative (25% acetic acid in methanol) on glass covers. After digestion with pepsin for 15 min and dehydration with ethanol, probe mixture was applied. Probe denaturation during 75 °C for 3 min was followed by overnight hybridization at 37 °C in a humidified chamber. Post-hybridization washing was carried out in 0.4 × SSC solution (Life Technologies) at 73 °C for 2 min, and 1 min in 2 × SSC/0.1% NP-40 (Sigma-Aldrich) at room temperature. After mounting with Vectashield with 4',6-diamidino-2-phenylindole (Vector Labs, Brussels, Belgium), slides were analysed blindly and by two independent operators, using a Zeiss axyoplan-2 microscope. Statistics Fisher’s exact test was used for comparison of fractions of abnormal and normal cells derived from the aCGH and FISH data. Accession Codes : All array data are available at the Gene Expression Omnibus repository ( http://www.ncbi.nlm.nih.gov/gds ) with accession number GSE51126 . How to cite this article: Jacobs, K. et al . Low-grade chromosomal mosaicism in human somatic and embryonic stem cell populations. Nat. Commun. 5:4227 doi: 10.1038/ncomms5227 (2014).